Ray-optics cloaking devices for large objects in incoherent natural light A cloak that can hide living creatures from sight is a common feature of mythology but still remains unrealized as a practical device. To preserve the wave phase, the previous cloaking solution proposed by Pendry and colleagues required transformation of the electromagnetic space around the hidden object in such a way that the rays bending around the object inside the cloak region have to travel faster than those passing it by. This difficult phase preservation requirement is the main obstacle for building a broadband polarization-insensitive cloak for large objects. Here we propose a simplified version of Pendry’s cloak by abolishing the requirement for phase preservation, as it is irrelevant for observation using incoherent natural light with human eyes, which are phase and polarization insensitive. This allows for a cloak design on large scales using commonly available materials. We successfully demonstrate the cloaking of living creatures, a cat and a fish, from the eye. Invisibility cloaking [1] , [2] , [3] , [4] , [5] , [6] , [7] , [8] , [9] , [10] , [11] , [12] , [13] , [14] , [15] , [16] , [17] , [18] was almost inconceivable until the ingenious theory of macroscopic invisibility cloaking was proposed based on transformation optics principles [2] , [3] . Because of the tremendous difficulty in practical realization, various approximations [4] , [5] , [6] , [19] were generally made to simplify the complexity of a perfect cloak. For example, non-magnetic optical cloaking was proposed by embedding metal nanowires in a dielectric material [5] . With these approximations, cloaks that could hide objects roughly one wavelength large (an optical wavelength equates to the scale of single-celled organisms) have been experimentally demonstrated in both the microwave [4] , [7] , [10] and optical spectrum [8] , [9] , [11] . Successful attempts have also been made to allow the cloaking technology to be used at much larger scales. The naturally anisotropic crystal of calcite has been used to realize invisibility at the scale of millimetres [12] , [13] for specifically polarized visible light in an environment of optical immersion oil. Developing a method of natural light cloaking in a natural environment at a scale sufficiently large for living creatures is a very challenging task. Recently, a significant step in this direction was reported: a microwave unidirectional cloak for a polarized wave in air successfully hid a freestanding object along a single direction with almost ideal performance; the object was approximately 10 wavelengths in length [18] . However, making a large-scale living creature invisible to the human eye has not yet been possible. In fact, all these difficulties in implementation stem from the need to bend light around the hidden object while preserving its phase. Indeed, the rays that go around the hidden object have longer physical paths. To preserve the phase, they need to travel much faster than other rays passing by the cloaking device, which subsequently leads to superluminal phase propagation and extreme material parameters [3] , [4] , [20] . The requirement of phase preservation is necessary at microwave frequencies because the phase of microwaves can be easily detected with an antenna. However, the premise of preserving the phase of light in a natural light optical cloaking device lacks rationale. Indeed, natural light is essentially randomly polarized and incoherent, and its phase is not well defined. Living creatures cannot sense the phase of light, and most of them, like humans, are largely insensitive to polarization. Therefore, abandoning the requirement of phase preservation for natural light cloaking makes it possible to hide large-scale living creatures. Here we demonstrate that by abandoning the phase preservation requirement, it is possible to create invisibility cloaking for natural light at multiple observation angles (see Supplementary Movies 1 and 2 documenting the real-life cloaking performance). Such a cloaking device operates within the ray-optics approximation. It will disregard the fine effects of interference seen in wave optics but will offer good performance for hiding macroscopic objects much larger than the wavelength of light. Recent theoretical developments in cloaking using non-Euclidean transformation [21] , [22] have provided an alternative method of abolishing phase preservation by incorporating anisotropic materials. Our experimental demonstration with only isotropic materials and incoherent light can serve as the first simplified test of a non-phase-preservation cloak. Compared with the previous unidirectional cloak design [18] , [19] , our method can be easily extended in multiple directions for arbitrary polarization over a broad range of optical frequencies, and therefore can significantly simplify the construction of a cloak in many real applications in which only a certain number of detectors or observers are involved. Using widely available optical glass, we constructed polarization-insensitive cloaks that were able to hide a fish in a fish tank and a cat in an ambient air environment. Design of a four-directional ray-optics square cloak We start with an analysis on how to simplify a perfect cloaking device designed by the transformation optics approach proposed by Pendry et al. [3] For comparison, we first analyse the case in which phase preservation is maintained, and later, we will abolish the phase preservation requirement. Consider a square cloaking device with a square ‘hole’ at the centre opened from coordinate transformation, as shown in Fig. 1a,b , in which horizontal rays propagate from left to right with their phase, or wavefronts, indicated with red dotted lines. In Fig. 1a , the virtual space with straight Cartesian coordinates represents an isotropic background medium with a relative permeability of μ b =1 and a relative permittivity of ε b . As the first step of simplification, an affine coordinate transformation is used to design the cloak such that the continuous inhomogeneity in the previous cloaking devices [3] , [4] can be avoided. Under this homogeneous coordinate transformation, the triangles OAB , OBC , OCD and ODA in the virtual space ( Fig. 1a ) are transformed to triangles FAB , GBC , HCD and EDA in the physical space ( Fig. 1b ), respectively. The lines AO , BO , CO and DO in the virtual space ( Fig. 1a ) are transformed to triangles AEF , BFG , CGH and DHE in the physical space ( Fig. 1b ), respectively. According to the principle of transformation optics [2] , [3] , the resultant square cloak with an inner radius of r 1 and outer radius of r 2 can be formed with two homogeneous and anisotropic materials, with their constitutive parameters expressed in their local coordinates as follows: (for material I , marked in green in Fig. 1b ), and (for material II , marked in pink in Fig. 1b ), where κ = r 2 cos( π /4)/[ r 2 cos( π /4)– r 1 ]. Compared with the previous cloak prototypes with inhomogeneous and anisotropic extreme material parameters [3] , [4] , the square cloak is simplified to one with only two homogeneous materials. 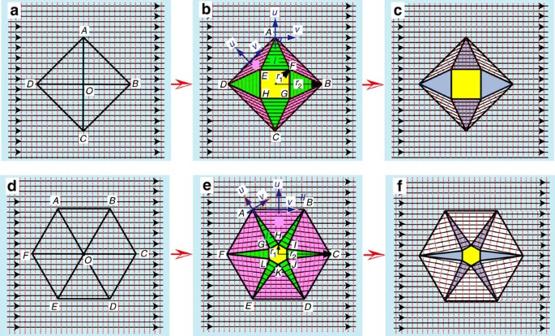Figure 1: Principle of natural light cloaking. Horizontal rays are incident from left to right. The red dotted vertical lines represent wavefronts when illumination is coherent. The central hidden region is marked in yellow. (a) The virtual space with straight Cartesian coordinates is filled with an isotropic background medium (marked in light blue) with a relative permeability ofμb=1 and a relative permittivity ofεb. The square in the virtual space is divided into four triangular sections and then transformed to the physical space by applying a homogeneous transformation in the local coordinates of each triangular section. (b) A perfect square cloak is designed by applying a coordinate transformation to open a square ‘hole’ at the centre. The wave has to propagate with infinite phase velocity in the singular anisotropic region (marked in green). (c) A four-directional square cloak with incident rays propagating horizontally. Wavefronts are perpendicular to the rays. (d) The hexagon in the virtual space is divided into six triangular sections and then transformed to the physical space by applying a homogeneous transformation in the local coordinates of each triangular section. (e) A perfect hexagonal cloak designed from coordinate transformation. (f) A six-directional hexagonal cloak with incident rays propagating horizontally. Wavefronts are perpendicular to the rays. Inbande, the cloaks require extreme and anisotropic material parameters. Incandf, the cloaks can be greatly simplified with isotropic materials while the invisibility performance is maintained in multiple directions. Figure 1: Principle of natural light cloaking. Horizontal rays are incident from left to right. The red dotted vertical lines represent wavefronts when illumination is coherent. The central hidden region is marked in yellow. ( a ) The virtual space with straight Cartesian coordinates is filled with an isotropic background medium (marked in light blue) with a relative permeability of μ b =1 and a relative permittivity of ε b . The square in the virtual space is divided into four triangular sections and then transformed to the physical space by applying a homogeneous transformation in the local coordinates of each triangular section. ( b ) A perfect square cloak is designed by applying a coordinate transformation to open a square ‘hole’ at the centre. The wave has to propagate with infinite phase velocity in the singular anisotropic region (marked in green). ( c ) A four-directional square cloak with incident rays propagating horizontally. Wavefronts are perpendicular to the rays. ( d ) The hexagon in the virtual space is divided into six triangular sections and then transformed to the physical space by applying a homogeneous transformation in the local coordinates of each triangular section. ( e ) A perfect hexagonal cloak designed from coordinate transformation. ( f ) A six-directional hexagonal cloak with incident rays propagating horizontally. Wavefronts are perpendicular to the rays. In b and e , the cloaks require extreme and anisotropic material parameters. In c and f , the cloaks can be greatly simplified with isotropic materials while the invisibility performance is maintained in multiple directions. Full size image However, the most challenging limitation for practical construction still remains in the regions marked in green in Fig. 1b , the wave needs to propagate with infinite phase velocity, which can be achieved only at a single frequency. Moreover, the extreme anisotropy, as derived in expressions of constitutive parameters in material I , requires the phase and ray to propagate perpendicularly to each other, which is practically difficult. To bypass this limitation of infinite phase velocity, in the second step of simplification, we consider only the rays propagating horizontally and rearrange their phase propagation in an attempt to reduce the complexity of practical construction. As a simple exercise, we rotate the phase lines to make them perpendicular to the ray lines and thus make the materials isotropic everywhere. After this simplification, the optical space perceived by the horizontal rays becomes the one in Fig. 1c . This optical space has inherited the invisibility performance from the original transformed cloak for horizontal rays. As a result, the cloak can be constructed without the need for metamaterials, using only isotropic and non-singular mediums. The requirement for infinite phase velocity is therefore removed. Because of its fourfold rotational symmetry, this simplified cloak can work for four different incident directions with arbitrary polarization. By selecting commonly available materials to fix the geometry, we can choose r 1 : r 2 =1:2.2, and subsequently, ε b : ε 1 : ε 2 =1.33 2 :1.83 2 :1. Here we have set the permeability in all regions equal to one and have rescaled the permittivities accordingly to keep the ray trajectories unchanged [4] , [5] , [12] , [13] . The resultant impedance mismatch will cause a slight reflection at the interfaces, which can be suppressed by practical antireflection techniques and thus is not considered here. Therefore, the cloak can be implemented with glass ( ε 1 =1.83 2 ) and air ( ε 2 =1) with a background of water ( ε b =1.33 2 ). The above example demonstrates the possibility of simplifying a perfect cloaking device using isotropic materials. However, because the phase preservation is still maintained, superluminal phase propagation is still required in the design unless the ambient medium possesses a refractive index higher than unity (such as water). Therefore, first, to achieve a broadband cloaking device in an air environment, we have to abolish the phase preservation requirement. Second, extending the cloaking performance in more directions (for example, six directions) using isotropic materials is almost impossible if phase preservation is required. In what follows, we will explore a more complex hexagonal cloak to demonstrate cloaking without phase preservation in ambient water and air. Design of a six-directional ray-optics hexagonal cloak Consider a perfect, phase-preserving omnidirectional hexagonal cloak designed by an affine coordinate transformation from the virtual space ( Fig. 1d ) to the physical space ( Fig. 1e ). The triangles OAB , OBC , OCD , ODE , OEF and OFA in the virtual space ( Fig. 1d ) are transformed to triangles HAB , IBC , JCD , KDE , LEF and GFA in the physical space ( Fig. 1e ), respectively, and the lines AO , BO , CO , DO , EO and FO in the virtual space ( Fig. 1d ) are transformed to triangles AGH , BHI , CIJ , DJK , EKL and FLG in the physical space ( Fig. 1e ), respectively. Therefore, similar to the perfect square cloak in Fig. 1b , a perfect hexagonal cloak with an inner radius of r 1 and outer radius of r 2 in Fig. 1e can be formed with two homogeneous and anisotropic materials whose constitutive parameters have the same expressions as the perfect square cloak, given that κ = r 2 cos( π /6)/[ r 2 cos( π /6)– r 1 ] in the case of the hexagonal cloak. The perfect hexagonal cloak ( Fig. 1e ) with extreme and anisotropic material parameters also requires the wave to propagate with infinite phase velocity and thus can be constructed using metamaterials only. To simply the construction, we can rotate the phase lines to rearrange the phase propagation and make all regions isotropic. Here when abolishing the phase preservation requirement, we still expect the transmitted rays to return to their original trajectories, whereas both the ray path and phase can be changed inside the cloak. We particularly choose the background to be water ( ε b =1.33 2 ) as the same to the previous simplified square cloak. In Fig. 1f , we choose r 1 : r 2 =1:5.26, and the required permittivities for the simplified hexagonal cloak are ε b : ε 1 : ε 2 =1.33 2 :1.78 2 :1. Again, the reflection at the interfaces between different regions is ignored. Figure 1f shows that the phase rearrangement causes wavefront dislocations in the simplified cloak. However, as will be demonstrated in the following sections, distortions caused by phase dislocations can be disregarded in experimental observations in incoherent natural light. Experimental characterization of the aquatic cloak Using the simplified sixfold cloaking design, we first construct a cloak hiding a fish in an aquatic environment using widely available optical glass. The cloak is constructed with six isosceles triangles of air with a refractive index of n 2 =1 and six isosceles triangles of glass with a refractive index of n 1 =1.78, as shown in Fig. 2a . The angle at the apex of the isosceles triangle of glass is α =13°, and the angle at the apex of the isosceles triangle of air is β = α +60°. The central hexagon area is the hidden region. The cloak has an outer radius of r 2 =60 mm, an inner radius of r 1 =11.4 mm and a height of h =50 mm. Analytical calculations show that the optical path length of the rays travelling through the cloak is 0.02 m shorter than the optical path length of those passing by the cloak. 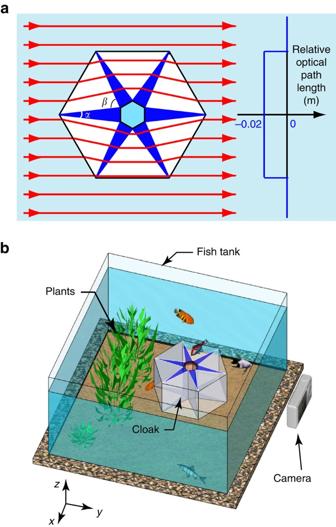Figure 2: Experimental fabrication and set-up of the aquatic ray cloak. (a) Ray diagram of light passing through the cloak in an aquatic environment. The background and the region in the centre (both are marked in light blue) contain water (nb=1.33). The region marked in white is air (n2=1). The region in dark blue is glass (n1=1.78) with an angleα=13°. The plot on the right shows the optical path length of the rays travelling through the cloak and those travelling straight in water (used as a reference). (b) Experimental set-up in a fish tank. The cloak is constructed with six pieces of glass withn1=1.78 (indicated in dark blue) enclosed in a hollow hexagonal container made of transparent glass. Figure 2b shows the experimental set-up in which a cloak is immersed in a fish tank filled with water with a refractive index of n b =1.33; the tank serves as a living environment for a goldfish. In the cloak fabrication, the outer shell of the cloak is constructed by gluing together thin glass pieces (with a thickness of 2 mm), a technique that is used to separate the background medium from the air space inside the cloak. Some green grass behind the cloak is used as background scenery to verify the performance of the cloak, and also to provide oxygen for the fish. A camera placed in front of the tank records the dynamic scene from the front observation angle. Figure 2: Experimental fabrication and set-up of the aquatic ray cloak. ( a ) Ray diagram of light passing through the cloak in an aquatic environment. The background and the region in the centre (both are marked in light blue) contain water ( n b =1.33). The region marked in white is air ( n 2 =1). The region in dark blue is glass ( n 1 =1.78) with an angle α =13°. The plot on the right shows the optical path length of the rays travelling through the cloak and those travelling straight in water (used as a reference). ( b ) Experimental set-up in a fish tank. The cloak is constructed with six pieces of glass with n 1 =1.78 (indicated in dark blue) enclosed in a hollow hexagonal container made of transparent glass. 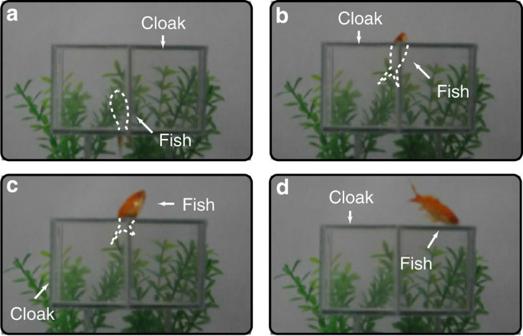Figure 3: Experimental observation of fish in the aquatic ray cloak. Dynamic monitoring of a fish swimming through the aquatic ray cloak. The outline of the invisible fish body is indicated by dotted lines. (a) The main fish body inside the cloak is invisible; only the tail outside of the cloak is visible. (b) Only the fish head outside of the cloak is visible. (c) The main body of the fish comes out of the cloak and thus becomes visible. (d) The whole fish has come out of the cloak. Full size image Figure 3a–d shows the dynamic process of the goldfish swimming from inside the cloak to the external aquatic environment. When swimming inside the cloak, the goldfish becomes invisible and does not block the scene of green plants behind the cloak. The edges of the transparent container are still visible because of some glue residue left at the edges of this homemade container. This cloak works for six different incident directions. Figure 3: Experimental observation of fish in the aquatic ray cloak. Dynamic monitoring of a fish swimming through the aquatic ray cloak. The outline of the invisible fish body is indicated by dotted lines. ( a ) The main fish body inside the cloak is invisible; only the tail outside of the cloak is visible. ( b ) Only the fish head outside of the cloak is visible. ( c ) The main body of the fish comes out of the cloak and thus becomes visible. ( d ) The whole fish has come out of the cloak. Full size image Experimental characterization of the terrestrial cloak Now we proceed to extend the simplified cloak from the aquatic environment to a terrestrial one with air as the ambient medium. We could put prisms around the cloak designed in Fig. 1c to construct a four-directional cloak in air. However, for simplicity of demonstration, we construct a unidirectional cloak instead that can hide terrestrial creatures from forward and backward observation angles. We use a cat as the terrestrial creature in the experiment. The cloak is constructed with four isosceles triangles and four right-angle triangles of the same glass material with a permittivity of ε 1 =1.78 2 . As only one direction is important, the original left and right isosceles triangles in the model of Fig. 1f are removed. The other regions are just air. When light propagates along the horizontal direction, the cloak can guide the light around the central hidden region and return them to the original paths at the other side of the cloak. The cloak designed for the terrestrial creatures is 0.07 m high, 0.3 m long and 0.26 m wide. 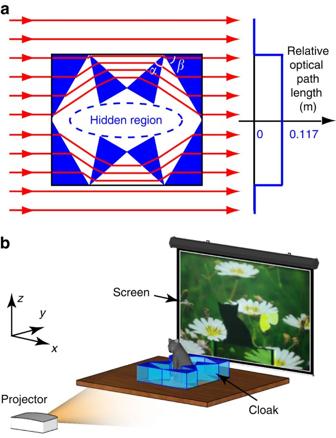Figure 4: Experimental fabrication and set-up of the terrestrial ray cloak. (a) Ray diagram of light passing through the cloak in a terrestrial environment. The region in dark blue is glass (n1=1.78). The other regions marked in white are air (nb=1). The angles of the pieces of glass areα=36.5° andβ=60°. The cloak is 0.3 m long, 0.26 m wide and 0.07 m high. The plot on the right shows the optical path length of the rays travelling through the cloak and those travelling straight in air (used as a reference). (b) Experimental set-up to test the cloaking performance. An office projector projects a movie through the cloak onto the screen behind the cloak. A camera (not shown here) placed behind the screen records the movie on the screen. A live cat is sitting inside the cloak. The width of the hidden area is approximately w =0.126 m. Figure 4a shows the ray tracing of the light incident onto the cloak and the optical path length of the rays transmitted from one side to the other side. The rays going through the cloak have travelled a longer optical path length than those passing by the cloak. Figure 4: Experimental fabrication and set-up of the terrestrial ray cloak. ( a ) Ray diagram of light passing through the cloak in a terrestrial environment. The region in dark blue is glass ( n 1 =1.78). The other regions marked in white are air ( n b =1). The angles of the pieces of glass are α =36.5° and β =60°. The cloak is 0.3 m long, 0.26 m wide and 0.07 m high. The plot on the right shows the optical path length of the rays travelling through the cloak and those travelling straight in air (used as a reference). ( b ) Experimental set-up to test the cloaking performance. An office projector projects a movie through the cloak onto the screen behind the cloak. A camera (not shown here) placed behind the screen records the movie on the screen. A live cat is sitting inside the cloak. Full size image To decisively demonstrate the capability of this cloaking strategy to hide creatures, especially with a dynamic background under natural light illumination, we use an office projector equipped with an incandescent bulb to project dynamic field scenery through the cloak ( Fig. 4b ). The light emitted from the incandescent bulb has very similar characteristics to natural light in terms of random polarization, incoherence and a continuous visible spectrum. A screen behind the cloak is used to display the projected image. Video recordings illustrating the cloak performance can be found in Supplementary Movies 1 and 2 . 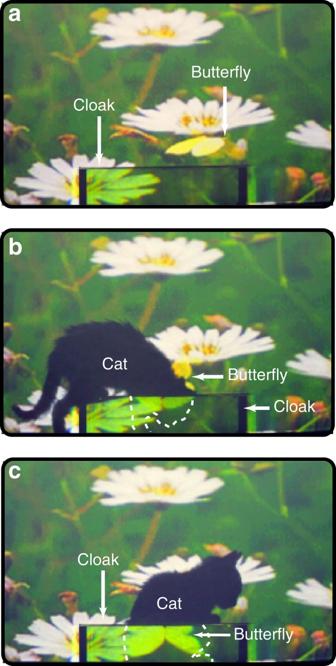Figure 5: Experimental observation of a cat in the terrestrial ray cloak. (a–c) The images displayed on the screen when (a) only the cloak is present, (b) a live cat is stepping into the cloak and (c) the main body of the cat has settled inside the cloak. The outline of the invisible body of the cat is indicated by dotted lines. During the whole process, the butterfly in the background scenery is moving. Figure 5a–c shows pictures on the screen captured by a digital camera behind the screen. Figure 5a shows an image in which only the cloak is present in front of the background scenery where a yellow butterfly is flitting among flowers. The cloak casts some moderate edge shadows because the light coming from the projector is divergent rather than being ideally parallel. In Fig. 5b , a living cat is stepping into the cloak. One can see clearly that the head and forelegs of the cat inside the cloak become invisible. In Fig. 5c , the main body of the cat has settled inside the cloak and becomes invisible, whereas the head and forelegs of the cat outside the cloak are still visible and block the white flower in the middle. At this moment, the projected butterfly is flitting quickly from the upper left to the lower right behind the cloak but still can be seen clearly on the screen through the body of the cat. Figure 5: Experimental observation of a cat in the terrestrial ray cloak. ( a – c ) The images displayed on the screen when ( a ) only the cloak is present, ( b ) a live cat is stepping into the cloak and ( c ) the main body of the cat has settled inside the cloak. The outline of the invisible body of the cat is indicated by dotted lines. During the whole process, the butterfly in the background scenery is moving. Full size image Cloaking tolerance for oblique viewing angles The above cloaks are designed for certain discrete angles. To complete the analysis, we also characterize sensitivity of the cloaking performance for oblique viewing angles. To facilitate comparison, we fix the camera and the background scenes at their physical positions but rotate the cloaks to change viewing angles from 0° to 5°. The results for the aquatic cloak are shown in Fig. 6 . One can see that when the angle varies between −2° and +2°, the image distortion captured by the camera is very small, indicating that the cloaking performance is still reasonably valid when viewed from a slightly oblique angle. When the angle increases further, for example, from +3° to +5° or from −3° to −5°, one can see that the image distortion becomes noticeable. Owing to the sixfold symmetry of the cloak, the cloaking performance can tolerate an angle variation of ~4° for every 60°. 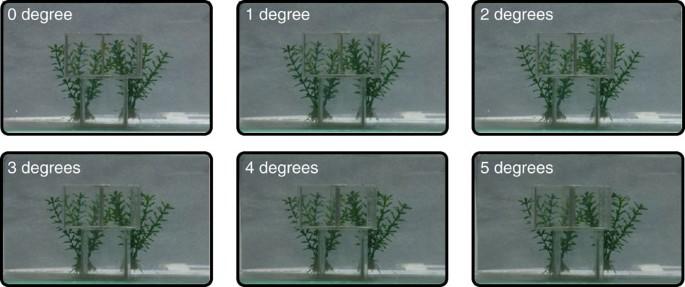Figure 6: Characterization of the aquatic cloak for different observation angles. The observation angle varies from 0° to 5° continuously as the image distortion changes from unnoticeable to noticeable. Figure 6: Characterization of the aquatic cloak for different observation angles. The observation angle varies from 0° to 5° continuously as the image distortion changes from unnoticeable to noticeable. Full size image Similarly, Fig. 7 shows the results for the unidirectional terrestrial cloak. From the results, one can see that when the light is normally incident on the cloak, that is, 0° incidence, the hidden region causes no shadow. When the incident angle increases from 0° to±2°, the hidden region starts to cast a thin shadow that is much smaller than the size of the hidden region (about half the width of the cloak), indicating that the cloak can still significantly reduce the cross-section of the hidden region. When the incident angle increases to±5°, the shadow becomes comparable to the size of the cloak and the image distortion becomes significant. Therefore, the performance of the terrestrial cloak is still acceptable in the range from −2° to 2°. 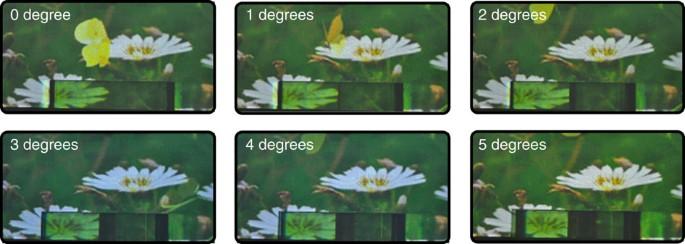Figure 7: Characterization of the terrestrial cloak for different observation angles. The observation angle varies from 0° to 5° continuously as the image distortion changes from unnoticeable to noticeable. Figure 7: Characterization of the terrestrial cloak for different observation angles. The observation angle varies from 0° to 5° continuously as the image distortion changes from unnoticeable to noticeable. Full size image Our demonstration of large-scale invisibility cloaking in multiple directions shows that cloaking is possible without using sophisticated engineered metamaterials. Our work also uniquely demonstrates a potential route towards large-scale omnidirectional invisibility, which so far has only existed in theory. Although the demonstrated cloaking solution is only effective for several observation directions, our work has successfully demonstrated the potential for practical applications of invisibility cloaking in hiding large-scale creatures in plain sight. By reconfiguring the prisms, the cloak operators could make them disappear from sight along any given direction, which would be important for security, entertainment and surveillance applications. For example, a ray-optics cloak mounted with a pinhole camera that can monitor the observer can rotate its cloaking direction towards the observer to make itself disappear from sight. Recently, reconfigurable or actively controllable cloaking technology [17] has emerged as a powerful strategy that allows dynamical optimization of the cloaking performance based on feedback from the external environment. We expect our work will be more applicable when control strategies are integrated. How to cite this article: Chen, H. et al. Ray-optics cloaking devices for large objects in incoherent natural light. Nat. Commun. 4:2652 doi: 10.1038/ncomms3652 (2013).